Integrable microwave filter based on a photonic crystal delay line The availability of a tunable delay line with a chip-size footprint is a crucial step towards the full implementation of integrated microwave photonic signal processors. Achieving a large and tunable group delay on a millimetre-sized chip is not trivial. Slow light concepts are an appropriate solution, if propagation losses are kept acceptable. Here we use a low-loss 1.5 mm-long photonic crystal waveguide to demonstrate both notch and band-pass microwave filters that can be tuned over the 0–50-GHz spectral band. The waveguide is capable of generating a controllable delay with limited signal attenuation (total insertion loss below 10 dB when the delay is below 70 ps) and degradation. Owing to the very small footprint of the delay line, a fully integrated device is feasible, also featuring more complex and elaborate filter functions. M icrowave photonics (MWPs) [1] , [2] , [3] , which brings together the worlds of radiofrequency engineering and optoelectronics, has attracted great interest from both the research community and the commercial sector over the past 30 years, and is set to have a bright future [4] . Its benefit stems from the fact that it enables the realization of key functionalities in microwave systems that are either complex or even not directly possible in the radio frequency (RF) domain. An important example is microwave signal filtering, which is ubiquitous in communications, radio-over-fibre, radar, radio astronomy and digital satellite communication systems [5] . Agility, reconfiguratibily and tunability are highly desirable features, which are, however, not straightforward to implement using traditional electronic circuitry, for example, microstrip [6] or coplanar waveguide lines [7] , substrate-integrated waveguides [8] and superconducting circuits [9] . To this end, approaches based on ferroelectric materials are being investigated, such as barium strontium titanate [10] , semiconductor varactors diodes [6] , metamaterials [7] , micro-electro-mechanical systems [8] and SiGe BiCMOS-compatible structures [11] . However, only MWP approaches have provided, to date, promising results in terms of tunability, reconfigurability and broadband operation. MWP signal processors reported so far [12] , [13] , [14] , [15] , [16] have relied on discrete optoelectronic devices and standard optical fibre delay lines, and components leading to bulky, expensive and power-consuming architectures. Typical delay line footprints range from several tens of centimetres when using fibre Bragg gratings (FBGs) to a few kilometres when using standard optical fibres. A solution to the above limitations of MWP filters is contingent on the possibility of incorporating this functionality into an application-specific photonic integrated circuit, which makes the former approaches based on extended delay lines inapplicable. Preliminary efforts towards integration have relied on resonant delay lines provided by ring cavities and coupled resonant optical waveguides [17] , [18] , [19] , [20] . These approaches suffer from an intrinsic trade-off between dispersion and bandwidth, preventing broadband operation. Thus, the cornerstone towards the integration of MWP filters resides in the availability of an integrated delay line, suitably designed to operate with MWP signals and providing enough dispersion. In this context, photonic crystal (PhC) waveguides are potential candidates, as the dispersion profile can be tailored to an extent that is no match with other photonic structures [21] , [22] . In this work, we provide the first ever demonstration of tunable and reconfigurable MWP filters based on a 1.5-mm-long GaInP/GaAs highly dispersive PhC waveguide delay line optimized for RF signals. The reduced waveguide loss in the slow light regime, owing to both design and fabrication optimization, is crucial to achieve the large dispersion values required for the integrated delay line. The salient features include: notch and band-pass operation; a footprint reduced by several orders of magnitude compared to filters based on FBG or fibre delay lines; broadband operation up to 50 GHz; and tunable free spectral ranges over 70 GHz. In addition, there is clear potential for the improvement of the selectivity, the main to secondary side-lobe (MSSL) ratio and the Q factor, thereby leading to high-performance MWP filtering owing to compatibility with sources of optical frequency combs [23] . Basic concept The most powerful and versatile approach for the implementation of MWP filters is that based on incoherent discrete signal processing [24] . In particular, finite impulse response [5] filters combine at their output a finite set of delayed and weighted replicas or taps of the input optical intensity signal (a RF-modulated optical carrier) [5] . The usual implementation of this concept in the context of MWPs can follow two approaches as shown in Fig. 1 . In the first one ( Fig. 1a ), the delays set to multiples of T are obtained, for instance, by means of a set of N non-dispersive optical fibre coils where the length of the fibre in the k -th tap is c ( k−1 ) T/n , where c is the light velocity in the vacuum and n is the refractive index. This simple scheme does not allow tuning, as this would require changing the value of T . An alternative approach ( Fig. 1b ) is based on the combination of a dispersive delay line and different optical carriers. Here the optical sources emit at different wavelengths so the spectral separation of a pair of consecutive modes implementing consecutive taps is Δλ , and the basic delay is given T = DLΔλ , where L represents the length of the dispersive element and D its dispersion parameter. Thus, the value of the basic delay T is changed by tuning the wavelength separation among the carriers, thereby allowing tunability [25] . Although in the first case the intensity or weight a k of the k -th tap can be changed by inserting loss/gain devices in the fibre coils, with the second approach, a k is readily adjusted by changing the optical power emitted by the optical sources [12] , [25] . In this work, we focus on the approach of Fig. 1b , as it is more flexible. 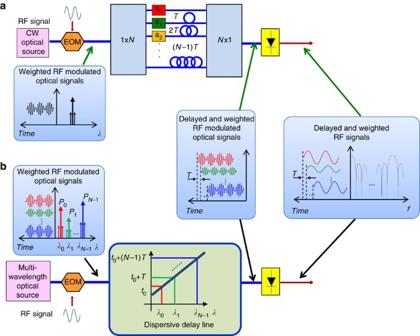Figure 1: General schematics of a MWP multi-tap filter. (a) Traditional approach based on a single optical source in combination with multiple non-dispersive short fibre coils. The basic delayTis implemented by means of a dispersionless fibre coil of lengthcT/n, wherecstands for the speed of light in vacuum andnis the refractive index of the core. The RF-modulated optical signal is divided by a 1×Ncoupler intoNtaps or samples. The weight of each sample can be changed by means of an individual attenuator or amplifier. For instance, thek-th tap is weighted in power by the attenuator/amplifier providing a value ofakand it is delayed by (k−1)Tby means of a fibre coil of length (k−1)cT/n. The signal samples are combined by means of aN×1 coupler and fed to the photodetector. The boxes connected with green arrows show the time and frequency domain structure of the signals at selected points of the layout. (b) A more compact approach based on a multi-wavelength optical source together with a single dispersive element. The optical sources emit at different wavelengths so the spectral separation of a pair of consecutive modes implementing consecutive taps isΔλ, and their basic delay is given byT=DLΔλwhereLrepresents the length of the dispersive element andDits dispersion parameter. Here, the intensity or weightakof thek-th tap can be adjusted by changing the optical power emitted by the optical sources. The boxes connected with black arrows show the time and frequency domain structure of the signals at selected points of the layout. Figure 1: General schematics of a MWP multi-tap filter. ( a ) Traditional approach based on a single optical source in combination with multiple non-dispersive short fibre coils. The basic delay T is implemented by means of a dispersionless fibre coil of length cT/n , where c stands for the speed of light in vacuum and n is the refractive index of the core. The RF-modulated optical signal is divided by a 1× N coupler into N taps or samples. The weight of each sample can be changed by means of an individual attenuator or amplifier. For instance, the k -th tap is weighted in power by the attenuator/amplifier providing a value of a k and it is delayed by ( k −1 )T by means of a fibre coil of length ( k −1) cT/n . The signal samples are combined by means of a N ×1 coupler and fed to the photodetector. The boxes connected with green arrows show the time and frequency domain structure of the signals at selected points of the layout. ( b ) A more compact approach based on a multi-wavelength optical source together with a single dispersive element. The optical sources emit at different wavelengths so the spectral separation of a pair of consecutive modes implementing consecutive taps is Δλ , and their basic delay is given by T = DLΔλ where L represents the length of the dispersive element and D its dispersion parameter. Here, the intensity or weight a k of the k -th tap can be adjusted by changing the optical power emitted by the optical sources. The boxes connected with black arrows show the time and frequency domain structure of the signals at selected points of the layout. Full size image Implementation of the PhC delay line A PhC waveguide results from a missing line in a regular lattice of holes on a self-standing dielectric (here GaInP) slab, as shown in Fig. 2a,b . Owing to the inherently complex waveguiding mechanisms originating from Bragg scattering in the photonic lattice, the dispersion of such waveguides departs from that of their more conventional counterparts, such as, for instance, rib-loaded structures. A decade ago, it was demonstrated that in a PhC waveguide the group velocity might vary from c /5 up to c /90, thereby laying the foundations of a chip-sized optical delay-line [21] . Since then, PhC waveguides have been intensively investigated for generating slow-light [26] . 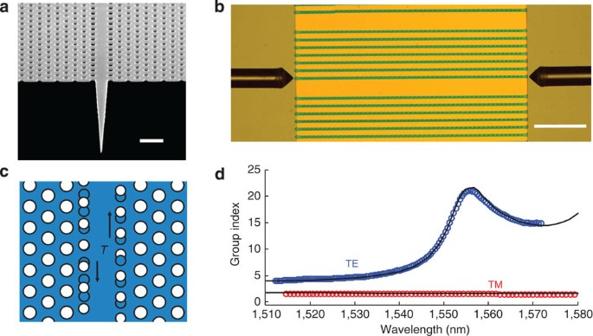Figure 2: PhC design. (a) SEM image of the tapered coupler at the end of the PhC waveguides (the scale bar is 1 μm). (b) Optical image of the chip containing the photonic crystal waveguides (green) and the coupling lensed fibres (the scale bar is 250 μm). (c) Design of the PhC waveguide with the anti-symmetric shift (of magnitudeT×a) of the first row of holes. (d) Measured (markers) and calculated (solid) dispersion (group index versus wavelength) for the TE and TM modes, showing good agreement. For details, see Methods. Figure 2: PhC design. ( a ) SEM image of the tapered coupler at the end of the PhC waveguides (the scale bar is 1 μm). ( b ) Optical image of the chip containing the photonic crystal waveguides (green) and the coupling lensed fibres (the scale bar is 250 μm). ( c ) Design of the PhC waveguide with the anti-symmetric shift (of magnitude T × a ) of the first row of holes. ( d ) Measured (markers) and calculated (solid) dispersion (group index versus wavelength) for the TE and TM modes, showing good agreement. For details, see Methods. Full size image Propagation loss in PhC waveguides can be as low as a few dB cm −1 (ref. 27 ). However, it systematically increases when the group velocity is reduced, because of the enhanced impact of the fabrication imperfections, mainly roughness at the etched interfaces. This has been preventing the achievement of large optical delays with moderate attenuation and, thereby, practical use for implementing functions in the domain of optical signal processing until very recently [28] . By engineering the field distribution of the propagation mode, O'Faolain et al . [29] have demonstrated a substantial reduction of backscattering and an improvement of the transmission of modes with group velocity smaller than c /30 in silicon-based PhCs. It has been pointed out [29] that the attenuation (dB) per delay (ns) is more appropriate than attenuation per distance (dB cm −1 ), when referring to delay lines. In this respect, a remarkable figure of 25 dB ns −1 has been reported [29] . Still, here it is implicitly assumed that this figure, measured in short (a few hundreds of micrometres) waveguides, can be extrapolated to any length. Indeed, the theory supports this claim for single mode, missing line defect PhC waveguides, so long the disorder is assumed random and with the same statistics all long the waveguide [30] . It must also be pointed out that the attenuation (measured or calculated) is defined as an average over a large number. These points must be considered when considering the actual use of these waveguides in applications. For application in MWPs, a tunable delay as large as 100 ps is needed, which implies the use of a long waveguide, for example, in the millimetre range. Thus, the probability of multiple coherent scattering events is much stronger relative to a shorter (for example, 100 μm) waveguide that is operated at the same group velocity. This results in distortion of the transmission spectrum [31] , [32] , even leading to sharp resonant peaks, even when the group index ( n g = c / v g ) is relatively small (~15). This is even more detrimental for applications than the mere (averaged) value of the attenuation. Furthermore, the fabrication of long PhC waveguides implies a mechanical displacement of the sample; each time the maximum writing area of the electron beam system (typically a few hundreds of micrometres) is reached. That might lead to 'dislocations' (similarly to crystals) in the PhC pattern, thereby altering the statistics of the disorder along the waveguide. For all these reasons, the suitability of a PhC waveguide as a delay line for MWPs must be assessed under more realistic conditions, as follows. First, the total insertion losses, including input and output coupling, must be considered relative to the actual time delay (for example, 100 ps), and not extrapolated. Second, the delay should be continuously tunable, for example, transmission should not change abruptly when changing the operating point of the device. Finally, the signal distortion, due to coherent multiple scattering, must be taken into account by characterizing the sample with a signal with realistic bandwidth. Here, we report the design, fabrication and characterization of an optical delay line based on a PhC waveguide that meets these requirements. The use of the PhC waveguide was reported for the first time [33] using a simple missing line defect PhC waveguide. The delay achieved there was a few tens of picoseconds, strongly distorted by Fabry–Perot interference due to reflections at the as-cleaved waveguide ends. The waveguide design is characterized by an anti-symmetric shift of the first row of holes [34] , [35] , [36] , as indicated in Fig. 2c (see details in Methods). This modification of the waveguide symmetry induces a coupling between the even and odd mode resulting in a 'hump'-shaped dependence of the group index on the wavelength (see Fig. 2d ). Details are discussed in Colman et al . [36] The group delays for both TE (defined as the E field parallel to the membrane and perpendicular to the direction of propagation) and TM modes have been measured with an interferometric technique (see Methods). The calculated dispersion for both TE and TM modes is also plotted, with excellent agreement. The fabricated device is 1.5 mm long and contains mode adapters [37] , as shown in Fig. 2a , owing to which the total insertion loss (minimum value at low group index) is reduced to about 7 dB (from fibre to fibre, including propagation in the waveguide and fibre/PhC coupling). In addition, undesirable Fabry–Perot fringes in the transmission spectra are removed, as apparent in Fig. 3a . The residual modulation results from multiple coherent scattering [31] . The corresponding group index is also plotted in the same figure. The important point here is the moderate (3.5 dB) optical transmission penalty, as the group velocity is reduced to c /14. Thus, a delay of 70 ps is achieved with total insertion loss 10 dB from fibre to fibre. 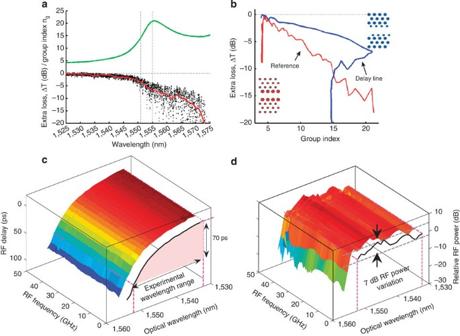Figure 3: Experimental characterization of the PhC waveguides. (a) Dispersion (group index versus wavelength, green solid line) and (red) excess transmission loss (that is, transmission normalized to maximum) of the TE even mode of the waveguide corresponding to the design with anti-symmetric shift (seeFig. 2c). The waveguide length is 1.5 mm. The vertical dashed lines correspond to the +3.5 and +7-dB extra-loss level and connect to the corresponding group index (14 and 21) and delay (~70 and 105 ps). (b) Excess loss versus the group index for the waveguide used for the delay line (blue, same data as inFig. 3a) compared with a reference sample with different design (red) used in the experiment by Roy35. (c,d) Measurements in the microwave domain of the sample referenced inFig. 2d. Relative delay (c) and power variation (d) of the microwave signal as a function of the wavelength of the optical carrier and the microwave frequency. Figure 3: Experimental characterization of the PhC waveguides. ( a ) Dispersion (group index versus wavelength, green solid line) and (red) excess transmission loss (that is, transmission normalized to maximum) of the TE even mode of the waveguide corresponding to the design with anti-symmetric shift (see Fig. 2c ). The waveguide length is 1.5 mm. The vertical dashed lines correspond to the +3.5 and +7-dB extra-loss level and connect to the corresponding group index (14 and 21) and delay (~70 and 105 ps). ( b ) Excess loss versus the group index for the waveguide used for the delay line (blue, same data as in Fig. 3a ) compared with a reference sample with different design (red) used in the experiment by Roy [35] . ( c , d ) Measurements in the microwave domain of the sample referenced in Fig. 2d . Relative delay ( c ) and power variation ( d ) of the microwave signal as a function of the wavelength of the optical carrier and the microwave frequency. Full size image We point out that not only the improvement of the fabrication process is important but also the choice of the waveguide design has a role. Figure 3b represents the transmission plotted against the group index. Two samples, fabricated within the same processing batch and only differing by the design, are compared. It is apparent that the design used for the delay line performs much better than the older design, represented with the red pattern. Consistently with the discussion above, we have assessed the performance of the PhC waveguide as a delay-line for microwave signals by measuring both the RF power and delay as a function of the wavelength of the optical carrier for the TE polarization mode (see Methods). The baseline used for the normalization was obtained by measuring the transfer function of the microwave link when the PhC was by-passed. The delay, which is defined as τ RF =d k /d ω and is plotted in Fig. 3c , involves the measurement of the microwave signal phase. Consistent with the interferometric measurements in Fig. 3a , a delay increase of 70 ps was achieved by sweeping the carrier wavelength from 1,532 to 1,552 nm. Besides, a flat response was obtained over the entire (0–50 GHz) RF frequency band of the microwave link, whatever the delay. The microwave bandwidth was limited by the measurement equipment (the modulator, detector and vector network analyzer (VNA)). Thereby, no appreciable signal degradation was introduced by the PhC waveguide. The amplitude transfer function is shown in Fig. 3d . A power variation of 7 dB, corresponding to a 3.5-dB change of the optical transmission, was experienced by the RF signal while tuning the delay by 70 ps, which is in perfect agreement with the optical transmission measurements described above. This figure guarantees a range of incremental delays between two different wavelengths, which is enough for filtering signals in the 10–100-GHz band. From the application standpoint, this change in amplitude, which can be easily compensated, is relatively small compared with other photonic approaches, particularly those based on resonant-type schemes. This point has considerable practical implications. The large bandwidth handling capability is a clear advantage. This large electrical bandwidth is still a small fraction of the optical transmission band (20 nm, hence about 3 THz), which explains why distortion can be reduced to a manageable level. Demonstration of filtering in the microwave domain In our simplest implementation of the filter on a PhC chip, we consider a two-tap MWP notch filter exploiting the group index disparity between the TE and TM modes. The principle is illustrated in Fig. 4a . The key point is that the dispersion of the TM is negligible when compared with the TE mode. Therefore, when the optical carrier is coupled to the two polarization modes, the modulation envelope experiences a relative delay between the TE and TM taps, which is controlled by the carrier wavelength. In addition, by properly adjusting the polarization state of the input optical signal, the relative weight of the two taps is also controlled. 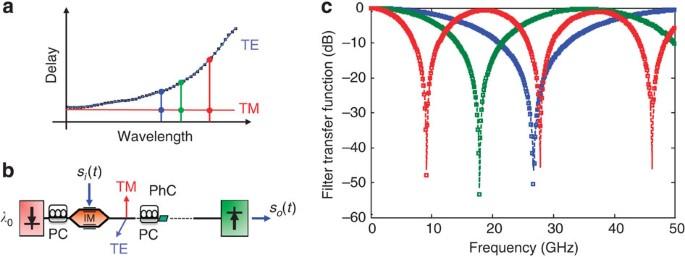Figure 4: Polarization-multiplex-based two-tap MWP filter. (a) The delay profiles, based on the experimental results obtained for the TE mode, for the TE and TM modes as a function of wavelength, for illustrative purposes of the filter operation. The TE and TM delays that correspond to the set of wavelengths selected for the filter experimental demonstration are indicated by colored dots, respectively, in blue, green and red for wavelengths of 1,544.5, 1,547 and 1,550.8 nm. (b) Experimental setup. A TLS emitting atλ0is modulated via a Mach–Zehnder modulator (IM) and carries the input electrical signalsi(t). A polarization controller is employed to optimize the power launched from the laser into the modulator. A second polarization controller ensures that both TE and TM polarizations are launched into the PhC. A photodetector then provides the output filtered electrical signalso(t). (c) Calculated (solid lines) and measured (squares) results for the filter response as a function of the wavelength. Blue, green and red markers, respectively, stand for 1,531, 1,537 and 1,542 nm optical wavelength. Figure 4: Polarization-multiplex-based two-tap MWP filter. ( a ) The delay profiles, based on the experimental results obtained for the TE mode, for the TE and TM modes as a function of wavelength, for illustrative purposes of the filter operation. The TE and TM delays that correspond to the set of wavelengths selected for the filter experimental demonstration are indicated by colored dots, respectively, in blue, green and red for wavelengths of 1,544.5, 1,547 and 1,550.8 nm. ( b ) Experimental setup. A TLS emitting at λ 0 is modulated via a Mach–Zehnder modulator (IM) and carries the input electrical signal s i ( t ). A polarization controller is employed to optimize the power launched from the laser into the modulator. A second polarization controller ensures that both TE and TM polarizations are launched into the PhC. A photodetector then provides the output filtered electrical signal s o ( t ). ( c ) Calculated (solid lines) and measured (squares) results for the filter response as a function of the wavelength. Blue, green and red markers, respectively, stand for 1,531, 1,537 and 1,542 nm optical wavelength. Full size image The generic layout of this polarization multiplexing PhC-based MWP filter is illustrated in Fig. 4b . The optical carrier, modulated by the microwave signal s i ( t ), is polarized to be coupled into both the TE and TM modes of the PhC waveguide. The output electrical signal s o ( t ), after propagation through the waveguide and photodetection, results from the incoherent superposition of the intensities of the TE and TM modes. The contribution carried by the TM mode experiences a group delay τ TM =L × n g,TM /c ( L is waveguide length), with n g,TM close to the effective index of the PhC slab, roughly ~2, weakly dependent on the wavelength of the optical carrier. Conversely, the signal carried by the TE mode is delayed by τ TE =L × n g,TE (λ)/c , with n g,TE spanning between 5 and 20 ( Fig. 2d ). The filtered electrical signal at the output of the photodiode is then: which corresponds, in the microwave frequency domain, to the filter transfer function H(f) : being f the microwave frequency and FSR the free spectral range of the filter, equal to c/ ( L ( n g,TE ( λ ) −n g,TM )). By combining these equations with the calculated and measured dispersion curves for the TE and TM modes in Fig. 2d , the expected response of the filter is readily obtained (see Fig. 4c ). Experimental results are in good agreement with the theory, particularly when the delay-line is operated with the group index below 10 (blue and green curves in Fig. 4c ). Besides, it must be pointed out that, whatever the target frequency of the filter, a notch depth of 50 dB is achieved. This is a clear benefit of the integrated nature of the delay line. A small deviation from the theory is observed at larger frequencies, corresponding to a decrease of the transmission minimum to 30 dB. This is related to the residual distortion of the transfer function ( Fig. 2d ), which makes it difficult to adjust the tap weights perfectly all over the RF domain. More precisely; if α is the ratio of the electrical power between the taps, the filter extinction ratio ER, or notch depth, is given by ER = (1+ α ) 2 / (1− α ) 2 . A 30-dB notch depth thus corresponds to a 0.6-dB RF power fluctuation in the RF frequency span, which is precisely what is measured from Fig. 2d . A more powerful configuration for band-pass filtering, in terms of the quality (Q)-factor and design flexibility, entails a larger number of taps. The straightforward implementation, which we have chosen here, consists of a single dispersive channel and multi-carriers optical source (for example, a comb or wavelength division multiplexing source), all modulated by the same microwave signal. This concept is illustrated in Fig. 5a and it was implemented using a long chirped FBG [25] with maximum length about 40 cm (ref. 12 ). Equivalent configurations use dispersive optical fibre links (DOFL), with lengths up to 20 km (ref. 38 ), or dispersion-compensating fibres (DCFs) [23] . 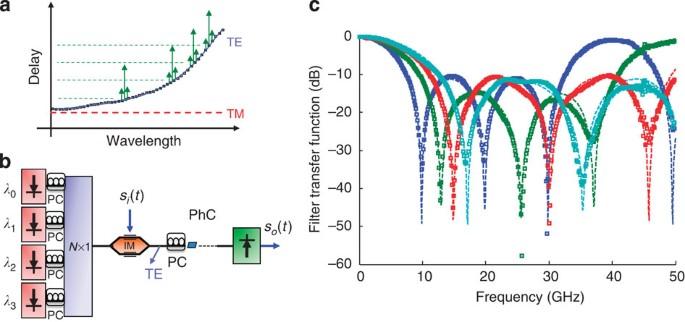Figure 5: Multi-wavelengh-based four-tap MWP filter. (a) The delay profiles, based on the experimental results obtained for the TE mode, for the TE and TM modes as a function of the wavelength for illustrative purposes of the filter operation. The green arrows show the spectral placement of the carriers and modulation sidebands (at 50 GHz) for all the four taps within the TE delay profile. This wavelength set is related to the green markers in figure (c), and corresponds to a constant group delay of 20 ps from tap to tap, which means a free spectral range of 50 GHz in the green filter transfer function in (c). (b) Experimental setup of the multi-wavelength filter. Four TLS (λ0toλ3) are combined and intensity modulated to carry the input electrical signalsi(t). The four wavelengths are then coupled into the photonic crystal delay line, along the TE mode, the RF delay for each tap being therefore a function of the tap wavelength. The polarization controllers perform the same functions as in the case of a single optical source. A photodetector provides the output filtered electrical signalso(t). (c) Calculated (dashed lines) and measured (colored squares) results for the filter response with different spectral scenarios of the emission wavelengths. The experimental wavelengths sets are 1,530, 1,546.4, 1,550.4, 1,552.6 nm (blue), 1,541.5, 1,548.9, 1,551, 1,552.7 nm (green), 1,545.2, 1,549.9, 1,551.2, 1,552.6 nm (red) and 1,546.8, 1,550.4, 1,551.5, 1,552.6 nm (cyan). Figure 5: Multi-wavelengh-based four-tap MWP filter. ( a ) The delay profiles, based on the experimental results obtained for the TE mode, for the TE and TM modes as a function of the wavelength for illustrative purposes of the filter operation. The green arrows show the spectral placement of the carriers and modulation sidebands (at 50 GHz) for all the four taps within the TE delay profile. This wavelength set is related to the green markers in figure ( c ), and corresponds to a constant group delay of 20 ps from tap to tap, which means a free spectral range of 50 GHz in the green filter transfer function in ( c ). ( b ) Experimental setup of the multi-wavelength filter. Four TLS ( λ 0 to λ 3 ) are combined and intensity modulated to carry the input electrical signal s i ( t ). The four wavelengths are then coupled into the photonic crystal delay line, along the TE mode, the RF delay for each tap being therefore a function of the tap wavelength. The polarization controllers perform the same functions as in the case of a single optical source. A photodetector provides the output filtered electrical signal s o ( t ). ( c ) Calculated (dashed lines) and measured (colored squares) results for the filter response with different spectral scenarios of the emission wavelengths. The experimental wavelengths sets are 1,530, 1,546.4, 1,550.4, 1,552.6 nm (blue), 1,541.5, 1,548.9, 1,551, 1,552.7 nm (green), 1,545.2, 1,549.9, 1,551.2, 1,552.6 nm (red) and 1,546.8, 1,550.4, 1,551.5, 1,552.6 nm (cyan). Full size image The same concept is here implemented by replacing the FBG/DOFL/DCF with an integrated PhC dispersive waveguide, thereby reducing the footprint of the key optical component by two orders of magnitude as compared with the FBG and six orders of magnitude as compared with the DOFL case. The layout of the four-tap PhC-based MWP filter (see Fig. 5b ) consists of four tunable lasers followed by a common modulator. The four replicas of the microwave signal are coupled into the TE mode of the PhC waveguide and, upon propagation, experience different delays, set to form uniform time intervals Δ τ by a suitable choice of the carrier wavelengths. As the carriers are not correlated together, the detected electrical signal is the incoherent sum of the optical intensities of the four paths and the corresponding transfer function in the microwave filter is: where FSR= 1/ Δ τ , and a k are the tap weights, adjusted by controlling the relative intensities of the tunable lasers. In the experimental demonstration reported here, all the filter taps a k were set to the same power level (that is, uniformly apodized filter), but variation of coefficients, leading to transfer function reconfiguration, is straightforward [5] . Hence, with a single tunable delay line with a maximum delay τ max and N taps, the FSR can be tuned from ( N −1) /τ max to infinity. The experimental result is reported in Fig. 5c and it is in very good agreement with the model. As we limited the group delay to 80 ps, spectral range of the filter is adjusted from 40 to 70 GHz. The maximum extinction ratio is 50 dB, whereas the MSSL ratio is about 10 dB. This figure can be improved by increasing the number of channels; however, at the expense of the lower bound of the tuning range. The distortion of the RF signal is very low over a broad spectral range (0–50 GHz). Towards integration With the demonstration of the suitability of a PhC waveguide as a delay line for microwave devices, all the key functionalities of the experimental setup described Fig. 5 could now be assembled in an integrated device. Indeed, optical modulators, photodetectors, splitters/combiners and laser sources are now available in integrated photonics platforms. In particular, integrated tunable laser sources (TLS) have recently been demonstrated on a silicon platform, through hybrid integration, which exhibit 45 nm tuning range around 1.5 μm. Alternatively, a similar tunability has been achieved on an InP platform with 13 dBm output power when followed by a co-integrated semiconductor optical amplifier (SOA) [39] . High-speed intensity modulation on a silicon platform has also been extensively studied in the past years and is still a very active topic. Modulation of 40 Gb s −1 has recently been achieved within the Helios project consortium with a Mach–Zehnder type device [40] . The electro-absorption modulators in germanium PIN on SOI (silicon on insulator) also exhibit interesting features of high bandwidth (up to 30 GHz), small footprint (a few tens of microns in length), low insertion loss (less than 5 dB) and extinction ratio up to 7 dB (ref. 41 ). Fast (bandwidth >40 Gb s −1 ) and efficient (responsivity=0.8A W −1 ) photodetectors have also been demonstrated on the same platform (germanium on SOI) [42] . Thus, the availability of a low-loss and tunable delay line, providing a large RF bandwidth, as demonstrated here, would complete the toolbox for the full integration of a MWPs filter. A possible layout representing the integrated counterpart of the experiment described above is shown in Fig. 6 . 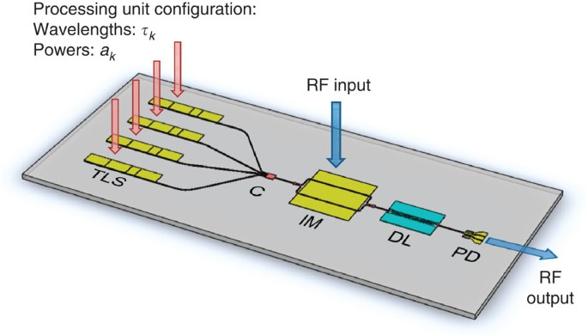Figure 6: Layout of a fully integrated microwave photonics signal processor. The weighting coefficientsakof the impulse response of the processing unit are programmed through the relative power levels of the TLSs, whereas the selected wavelengths set the taps group delaysτk, and hence the filter FSR. DL, photonic crystal delay line; IM, intensity modulator; PD, photodiode; Semiconductor optical amplifiers C, 4:1 optical combiner; TLS, tunable laser source. Figure 6: Layout of a fully integrated microwave photonics signal processor. The weighting coefficients a k of the impulse response of the processing unit are programmed through the relative power levels of the TLSs, whereas the selected wavelengths set the taps group delays τ k , and hence the filter FSR. DL, photonic crystal delay line; IM, intensity modulator; PD, photodiode; Semiconductor optical amplifiers C, 4:1 optical combiner; TLS, tunable laser source. Full size image Beyond the issue of manufacturability, the prospective integrated device must be analyzed with respect to the expected performances, in particular the power budget of the entire microwave link. In a photonic microwave device, this scales as the square of the total optical losses and as the square of the efficiency of the electro-optic intensity modulator. According to the literature, a 4:1 power combiner (for example, multimode interference coupler) and the intensity modulation (including insertion losses and bias point losses) exhibit cumulated optical losses in the range of 8 dB [43] , [44] . Including the PhC delay line, one ends up with ~15 dB of total optical losses (a more accurate estimate must take into account the on-chip coupling loss, likely smaller than fibre-PhC insertion losses). Thus, considering an optical power of 10 dBm at the output of each of the TLS, the RF power budget of the device (that is, the ratio between output and input RF power) is approximately −45 dB. This value is compatible with most practical system implementations. As a comparison, the power budget of a basic MWPs link (laser modulator fibre detector using discrete components) with 10 dBm optical power is already in the range of −25 dB. The PhCs-based filter is compared to other competing MWP implementations, as well as against purely electronic microwave devices. A summary of relevant results can be found in Table 1 . First, a single PhC waveguide enables a very large operating bandwidth, mainly limited by the disorder-induced distortion of the transmission, the bandwidth of the photodetectors and group velocity dispersion. The 50-GHz bandwidth reported here could be improved, through single-sideband modulation for instance. Although filters based on stimulated Brillouin scattering can achieve similar bandwidths, the integration is not possible and the power consumption (inherent to the stimulated Brillouin scattering effect) is large [45] , [46] . Power consumption is also a concern for filters based on SOAs [47] . Table 1 Comparison of the microwave filter with other technologies against the figures of merit. Full size table Because the proposed filter is based on a dispersive delay line, its performance can be affected by the power fading effect if double-sideband modulation is employed [1] , [2] , [3] . A straightforward measure to eliminate this limitation is to use single-sideband modulation [1] , [2] , [3] , which adds no significant complexity to the modulator. However, even if double sideband modulation is employed, the fact that the delay line length L is very small and that the power fading effect penalty is more severe the higher the product of the dispersion D and L is makes it possible to observe no significant penalty within the spectral range of interest. In our particular case, the power fading penalty was significant only above 80 GHz, which was outside our measurement range. The hybrid integrated approach [48] provides photodetector-limited bandwidth, combined with small footprint and very low loss. In addition, the tunability speed is very high. However, the tuning range is limited and the power consumption is not negligible as the structure integrates several active elements, such as SOAs. In terms of rejection level and bandpass/rejection bandwidth, the results reported here are still behind some of those achieved by using discrete component technologies. However, there is no fundamental limit to the improvement of these figures, rather, as the discrete filter is inherently scalable, the compactness of PhCs is an obvious advantage. In this implementation, the tuning speed depends on the optical source, which ultimately is limited by the carrier injection dynamics, namely in the nanosecond time scale. As 200 ns thermo-optical switching was demonstrated in PhC waveguides [49] , it is expected that our filter could be operated with a fixed wavelength source and tuned within comparable time scales. The bandpass width of our four-tap PhC-based filter is 8 GHz, which is adequate in the context of broadband signals processing, but could be improved depending on the number of taps. We point out that Supradeepa et al . [23] demonstrated a MWP filter based on a tailored optical comb source, combined with a DCF, with remarkable fast and broad tuning, high degree of reconfigurability and selectivity, owing to the large number of optical carriers used. The implementation of this design in our device is straightforward and would greatly benefit from the small footprint of the PhC delay line. A fully integrated device could be feasible. However, a linear dispersion profile is required as the frequency combs are equally spaced in frequency. In our device, the dispersion is nearly linear between 1,548 and 1,553 nm, with an average group velocity dispersion of ~10 ps nm −1 . If the frequency comb is spaced by 0.4 nm (~50 GHz), 12 optical carriers could be accommodated, resulting into a delay interval τ/( N –1) ≈4 ps, that is, the FSR is 250 GHz. A more appropriate design of the PhC delay line would improve this figure. Description of the figures of merit In bandpass filters, bandwidth is defined as the −3-dB or the full width half maximum of the passband, whereas for notch filters it refers to the spectral width at the rejection level of 20 dB with respect to the maximum. The operational bandwidth is defined as the spectral range within which the filter response can be tuned (it may not necessarily be equal to the spectral period or FSR). The central frequency refers, in the case of bandpass filters, to the position of the first maxima without considering baseband, whereas in notch-type filters, it corresponds to the frequency where the operational bandwidth centres. Size and insertion loss address here only the subsystem that enables filter tunability, that is, the delay line in our PhC-based filter implementation. In addition, insertion loss refers to the overall optical loss in MWP and electrical loss in MW filters. The rejection level indicates the MSSL ratio for bandpass filters, while it addresses the transmission minimum in the notch-type filters. The tunability range accounts for the FSR in both bandpass and notch-type filters. The lowest timing scale to perform filter tunability is given by the tunability speed. The power consumption only refers to the power required to operate the delay line. Here, 'high' indicates more than 100 mW, whereas 'medium' indicates a power consumption range in between 10 and 100 mW. PhC waveguide fabrication PhC waveguides were fabricated using a planar process. First, a 200-nm-thick mask of silica was deposited on a semiconductor structure containing a 180-nm-thick layer of InGaP grown by metal-organic chemical vapour deposition on GaAs. A poly(methyl methacrylate) (PMMA) resist was spun on it and exposed using e-beam writer. After etching of the silica mask, the III-V material was processed via inductively coupled plasma etching and finally a self-standing membrane was obtained by wet etching of the underlying layer of GaAs. The waveguide design is shown in Fig. 1c . The lattice period a is 482 nm, whereas the radius of the holes is 0.26 a . The first row of holes exhibits a slightly smaller radius (0.25 a ) and is shifted on opposite directions along the waveguide axis by 0.15 a . Calculation of the PhC dispersion We used our own implementation of the 3D finite differences in time domain method with periodic boundary conditions; with x the propagation direction of the Bloch mode and a the period of the PhC lattice. The size of the unit cell for the calculation was: a ×20 a ×6 a and the mesh resolution was down to a /20. The estimated relative accuracy in the frequency was better than 1/1000. PhC characterization The dispersion of the waveguide was measured using a TLS, which was swept over its entire spectral range (1,510–1,630 nm). The signal was then split to build up a Mach–Zehnder interferometer (MZI), with one of the arms containing the PhC waveguide. The two outputs of the MZI were fed to a balanced photodetectors (characterized by a trans-impedance gain of 10 5 ) and the differential signal was digitized with a 14-bit analog-to-digital converter. The wavelength was monitored with a reference interferometer. The resulting interferogram S ( f ), with f the optical frequency, was filtered using a Gaussian window centred at f j and Fourier-transformed to obtain the time-resolved transmission S j ( t ). The group delay t ( f j ) is defined as the peak of S j ( t ). MWP link characterization The delay introduced by the PhC waveguide and the corresponding loss were measured in the RF domain by inserting the device into a MWP link. The optical carrier of the MWP link was generated by a TLS. The RF signal was fed into the link through the RF input of a 50-GHz bandwidth Mach–Zehnder electro-optic modulator (MZM), which modulates the optical carrier intensity. The laser delivered 5 dBm optical power to the input of the MZM electro-optic modulator. Insertion losses of the MZM where 5 dB resulting in a 0-dBm input power to the polarization controller deployed to adjust the polarization state at the input of the PhC waveguide. Lensed fibres were used for input and output optical coupling. A high-speed photodetector was followed by an RF amplifier to compensate for the loss introduced by the MZM and the PhC device. The resulting MWP link was characterized as a two-port electrical component using a VNA whose output and input ports were, respectively, connected to the MZM RF input and the RF amplifier output. The S21 parameter measured by the VNA provided both the RF power and phase transfer function from 10 MHz to 50 GHz. The measurements given in Fig. 2c,d are referenced to a first acquisition performed at the lowest optical wavelength, corresponding to a fast propagation regime in the PhC waveguide. MWP filters characterization The results for the two-tap filter implementation shown in Fig. 4 were measured by deploying the same experimental setup used for the MWP link characterization. On the other hand, the output signal of four tunable lasers was optically coupled prior the MZM for obtaining the four-tap filter response illustrated in Fig. 5 . As the detuning is large with respect to the phase matching condition [50] , no significant nonlinear effects were observed in the PhC waveguide. How to cite this article: Sancho, J. et al . Integrable microwave filter based on a photonic crystal delay line. Nat. Commun. 3:1075 doi: 10.1038/ncomms2092 (2012).